A sugar phosphatase regulates the methylerythritol phosphate (MEP) pathway in malaria parasites Isoprenoid biosynthesis through the methylerythritol phosphate (MEP) pathway generates commercially important products and is a target for antimicrobial drug development. MEP pathway regulation is poorly understood in microorganisms. Here we employ a forward genetics approach to understand MEP pathway regulation in the malaria parasite, Plasmodium falciparum . The antimalarial fosmidomycin inhibits the MEP pathway enzyme deoxyxylulose 5-phosphate reductoisomerase (DXR). Fosmidomycin-resistant P. falciparum are enriched for changes in the PF3D7_1033400 locus (hereafter referred to as PfHAD1 ), encoding a homologue of haloacid dehalogenase (HAD)-like sugar phosphatases. We describe the structural basis for loss-of-function PfHAD1 alleles and find that PfHAD1 dephosphorylates a variety of sugar phosphates, including glycolytic intermediates. Loss of PfHAD1 is required for fosmidomycin resistance. Parasites lacking PfHAD1 have increased MEP pathway metabolites, particularly the DXR substrate, deoxyxylulose 5-phosphate. PfHAD1 therefore controls substrate availability to the MEP pathway. Because PfHAD1 has homologues in plants and bacteria, other HAD proteins may be MEP pathway regulators. Isoprenoids are the largest and most diverse class of biomolecules [1] . Isoprenoids perform essential cellular functions such as respiration (ubiquinone) and membrane localization of proteins (prenylation). There is considerable commercial interest in the production of isoprenoid-derived secondary metabolites as pharmaceuticals (for example, artemisinin and taxol) and biofuels. Isoprenoids are synthesized from two five-carbon precursor molecules, isopentenyl pyrophosphate and its isomer, dimethylallyl pyrophosphate. Two metabolically and enzymatically distinct pathways exist for the synthesis of isopentenyl pyrophosphate and dimethylallyl pyrophosphate. Archaea, fungi and animals utilize a mevalonate-dependent pathway. In contrast, plastid-containing eukaryotes and most bacteria use an alternate route that proceeds through the key metabolite methylerythritol phosphate (MEP) ( Fig. 1 ) (ref. 2 ). 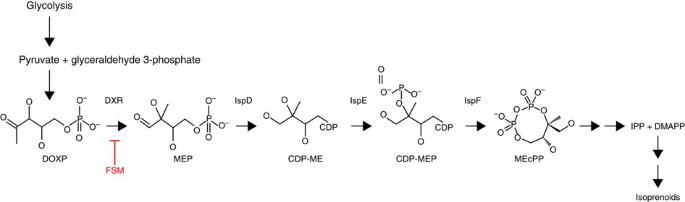Figure 1: The MEP pathway for isoprenoid biosynthesis. The MEP pathway for the synthesis of isoprenoids is specifically inhibited by FSM. FSM competitively inhibits PfDXR and indirectly inhibits PfIspD8. CDP-ME, 4-diphosphocytidyl-2-C-methylerythritol; CDP-MEP, 4-diphosphocytidyl-2-C-methyl-D-erythritol 2-phosphate; DMAPP, dimethylallyl pyrophosphate; DXR, DOXP reductase; IPP, isopentenyl pyrophosphate; IspD, CDP-ME synthase; IspE, CDP-ME kinase; IspF, MEcPP synthase. Figure 1: The MEP pathway for isoprenoid biosynthesis. The MEP pathway for the synthesis of isoprenoids is specifically inhibited by FSM. FSM competitively inhibits PfDXR and indirectly inhibits PfIspD [8] . CDP-ME, 4-diphosphocytidyl-2-C-methylerythritol; CDP-MEP, 4-diphosphocytidyl-2-C-methyl-D-erythritol 2-phosphate; DMAPP, dimethylallyl pyrophosphate; DXR, DOXP reductase; IPP, isopentenyl pyrophosphate; IspD, CDP-ME synthase; IspE, CDP-ME kinase; IspF, MEcPP synthase. Full size image In the MEP pathway, two glycolytic intermediates (glyceraldehyde 3-phosphate (gly3P) and pyruvate) are combined to generate deoxyxylulose 5-phosphate (DOXP) by DOXP synthase (DXS; E.C. 2.2.1.7). DOXP is subsequently reduced and isomerized to MEP in the first dedicated step of the MEP pathway, catalysed by deoxyxylulose phosphate reductoisomerase (DXR; E.C. 1.1.1.267). These first two steps of the MEP pathway are rate limiting in MEP-dependent isoprenoid biosynthesis [3] , [4] , [5] . Organisms may increase flux through the MEP pathway by increasing DXS and DXR production, or by increasing substrate availability for these enzymes [6] . The phosphonic acid antibiotic, fosmidomycin (FSM), competitively inhibits DXR in vitro [7] . Metabolic profiling of FSM-treated cells confirms that FSM inhibits MEP pathway metabolism within cells [8] . The growth effects of FSM are rescued by supplementation with downstream isoprenoids, confirming that the biological effects of FSM are mediated through isoprenoid biosynthesis inhibition [8] , [9] , [10] . These studies validate the use of FSM as a specific tool to probe the MEP pathway. Because chlorophyll biosynthesis requires MEP pathway-derived isoprenoids, FSM is a herbicide [11] . FSM resistance in the model plant, Arabidopsis thaliana , has been used to gain insight into MEP pathway regulation, and these studies have revealed post-transcriptional control of MEP pathway enzymes through an RNA metabolism protein (Rif10) (ref. 12 ). In contrast, there is little understanding of the MEP pathway regulation in non-model organisms. The malaria parasite, Plasmodium falciparum , depends on de novo isoprenoid biosynthesis through the MEP pathway [9] , [13] . Since drug resistance is one of the greatest challenges in malaria eradication, the MEP pathway is an attractive parasite-specific target for antimalarial drug development. As in plants, the MEP pathway in apicomplexan parasites is localized to a plastid-like organelle. The parasite organelle is called the apicoplast [14] , and isoprenoid synthesis may be the only required function of the apicoplast during blood-stage development [9] , [10] . Though not photosynthetic, the apicoplast shares a similar endosymbiotic origin with the plant chloroplast [15] . This uniquely positions P. falciparum in studies of MEP pathway biology as a plastid-containing eukaryote that is also a globally important pathogen. Here, to gain insight into how malaria parasites regulate isoprenoid precursor synthesis, we screen for P. falciparum strains able to survive MEP pathway inhibition by FSM. We uncover the first regulator of MEP pathway metabolism in malaria parasites, PF3D7_1467300 ( PfHAD1 ), a member of the haloacid dehalogenase (HAD) superfamily. Using detailed structural and biochemical studies, we show that FSM resistance is correlated with changes in PfHAD1 that ablate function. Further, we find that PfHAD1 is a cytosolic sugar phosphatase that dephosphorylates the intermediates of glycolysis. Loss of PfHAD1 function increases substrate availability to the MEP pathway and increases levels of isoprenoid precursors, thus conferring FSM resistance. Since close homologues of PfHAD1 are present in other MEP pathway-containing organisms, sugar phosphatases may represent a common strategy to regulate MEP pathway flux. Selection of FSM-resistant (FSM R ) P. falciparum The MEP pathway is essential for the synthesis of isoprenoids in P. falciparum [8] , [9] , [13] . The phosphonic acid antibiotic FSM specifically inhibits this pathway, primarily via competitive inhibition of PfDXR [7] ( Fig. 1 ). A FSM-sensitive 3D7 parental strain was subjected to FSM treatment at ~two to fourfold the wild-type half maximal inhibitory concentration (IC 50 ; Fig. 2a , Supplementary Table 1 ). This selection generated 19 independent FSM R strains of P. falciparum with increased IC 50 s for FSM ranging from 1.5–8.1 μM ( Fig. 2b , Supplementary Table 1 ). FSM R strains are also resistant to the related antibiotic, FR-900098 (ref. 16 ) ( Supplementary Fig. 1 ). 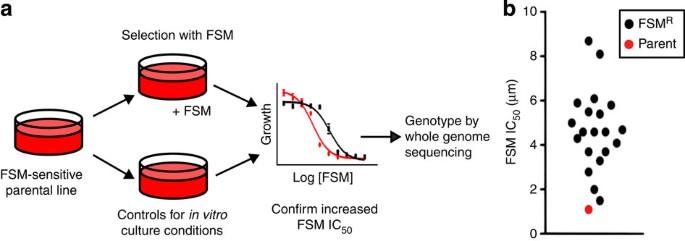Figure 2: Generation of FSM-resistant (FSMR)P. falciparum. (a) Schematic of selection of FSMRstrains. (b) FSMRstrains exhibit a range of resistance phenotypes. FSMRstrains have an average FSM IC50of 4.8±0.4 μM compared with the wild-type IC50of 1.1±0.2 μM. A complete list of strains and their IC50values are found inSupplementary Table 1. Figure 2: Generation of FSM-resistant (FSM R ) P. falciparum . ( a ) Schematic of selection of FSM R strains. ( b ) FSM R strains exhibit a range of resistance phenotypes. FSM R strains have an average FSM IC 50 of 4.8±0.4 μM compared with the wild-type IC 50 of 1.1±0.2 μM. A complete list of strains and their IC 50 values are found in Supplementary Table 1 . Full size image FSM resistance has been associated with copy number variations in the FSM target, PfDXR (PF3D7_1467300) (ref. 17 ). However, copy number changes that result in drug resistance often revert when selection is relieved [18] . To discourage PfDXR copy number variants, FSM R strains were cycled on and off drug treatment. All strains maintain their resistance phenotype after prolonged growth without FSM, and no changes in PfDXR transcript levels are observed in FSM R strains ( Supplementary Fig. 2 ). To control for genetic changes arising from prolonged culture or culture stresses, we performed control selections in which the parental 3D7 strain was cultured continuously for >3 months and, in some cases, was subjected to culture stresses such as depleted or incomplete media and aged (>90 days) erythrocytes. These strains retain their FSM sensitivity as measured by IC 50 (mean IC 50 1.8±0.4 μM). FSM R strains are enriched for genetic changes in PfHAD1 To uncover genetic changes correlated with FSM resistance, we genotyped the parent strain, six FSM R strains, and two control strains by whole genome sequencing with at least 15 × genome coverage. Sanger sequencing was used to verify single-nucleotide polymorphisms (SNPs) and insertion–deletions (indels) and to genotype loci of interest in strains whose genomes were not sequenced. We prioritized genetic changes found in coding regions and did not evaluate changes in highly variable loci (such as var and rifin genes) [19] , [20] . A list of SNPs uniquely identified in the FSM R strains is found in Supplementary Data 1 . The resulting data reveal a significant enrichment for nonsynonymous changes in PF3D7_1033400 in FSM R strains compared with control strains ( Fig. 3a ). We hereafter refer to PF3D7_1033400 as PfHAD1 . Fourteen of the 19 FSM R strains have a nonsynonymous change in PfHAD1 , while seven control laboratory strains do not have any sequence changes in PfHAD1 ( P =0.0012, Fisher’s Exact Test). 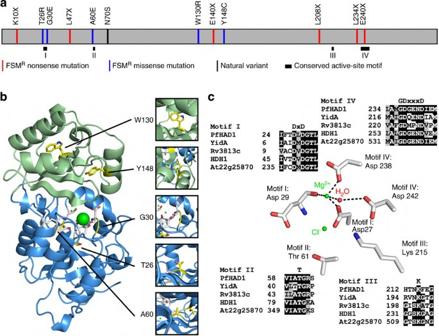Figure 3: FSMRvariants map to the core and active site regions of PfHAD1. (a) Schematic of PfHAD1 variants found in FSMRstrains. Six of the alleles result in premature stop codons. Five alleles produce full-length protein. N70S is a nondeleterious allele reported from sequenced clinical and laboratory isolates. Conserved active site motifs are shown as black boxes25. (b) Overall structure of PfHAD1 with the core domain in blue, cap domain in green and polymorphic residues mapped in yellow. Residues W130 and Y148 are located in the hydrophobic inner region of the cap domain. Residues T26 and A60 are located in the hydrophobic inner region of the core domain. Residue G30 is located in the substrate-binding site. (c) The backbone carbonyl oxygen of Asp-29 and the side chains of Asp-27 and Asp-238 coordinate a magnesium ion to form the active site. The side chains of Asp-29, Thr-61, and Lys-215 coordinate a chloride ion, and are correctly positioned to coordinate a phosphate group on substrate binding. These active-site residues are conserved inPfHAD1homologues from organisms possessing the MEP pathway. Alignment was produced in T-Coffee55using default parameters. Accession codes for NCBI protein sequences:E. coliYidA, EOU46719;M. tuberculosisRv3813c, NP_218330;C. reinhardtiiFER_156463, ADF43173;A. thalianaAt2g25870, ABO38782. Figure 3: FSM R variants map to the core and active site regions of PfHAD1. ( a ) Schematic of PfHAD1 variants found in FSM R strains. Six of the alleles result in premature stop codons. Five alleles produce full-length protein. N70S is a nondeleterious allele reported from sequenced clinical and laboratory isolates. Conserved active site motifs are shown as black boxes [25] . ( b ) Overall structure of PfHAD1 with the core domain in blue, cap domain in green and polymorphic residues mapped in yellow. Residues W130 and Y148 are located in the hydrophobic inner region of the cap domain. Residues T26 and A60 are located in the hydrophobic inner region of the core domain. Residue G30 is located in the substrate-binding site. ( c ) The backbone carbonyl oxygen of Asp-29 and the side chains of Asp-27 and Asp-238 coordinate a magnesium ion to form the active site. The side chains of Asp-29, Thr-61, and Lys-215 coordinate a chloride ion, and are correctly positioned to coordinate a phosphate group on substrate binding. These active-site residues are conserved in PfHAD1 homologues from organisms possessing the MEP pathway. Alignment was produced in T-Coffee [55] using default parameters. Accession codes for NCBI protein sequences: E. coli YidA, EOU46719; M. tuberculosis Rv3813c, NP_218330; C. reinhardtii FER_156463, ADF43173; A. thaliana At2g25870, ABO38782. Full size image Eleven alleles were represented in the 14 strains with PfHAD1 changes. Of these alleles, four indels and two nonsynonymous substitutions result in a truncated amino acid sequence ( Supplementary Table 1 ). The remaining five alleles are nonsynonymous substitutions that result in single amino acid changes. Four of these alleles are predicted to have deleterious effects on protein function by Polyphen-2, an algorithm for predicting the probability of functional effects of missense mutations (Polyphen-2 score >0.9) [21] ( Supplementary Table 1 ). Overall, FSM R strains are significantly enriched for likely deleterious changes in PfHAD1 , a previously uncharacterized gene, compared with FSM-sensitive control strains. In addition to the 3D7 PfHAD1 allele that we designate as wild-type, a nonsynonymous N70S variant has also been reported in sequenced clinical and laboratory isolates of P. falciparum [22] , [23] . This allele is not predicted to be deleterious (Polyphen-2 score=0.007). Two strains that possess the N70S allele, HB3 and Dd2, are not resistant to FSM (FSM IC 50 s of 1.3±0.2 μM and 0.6±0.09 μM, respectively). Five additional strains whose sequence data are available on public databases (7G8, D10, GHANA1, K1 and V1_S, plasmodb.org, accessed 4 November 2013) also possess the N70S allele. The minimal sequence variation in this gene in natural populations suggests that PfHAD1 has an important cellular function in P. falciparum . PfHAD1 is a Cof-like hydrolase member of the HAD superfamily Sequence homology places PfHAD1 in the HAD superfamily (Pfam PF08282) (ref. 24 ). Members of this large superfamily are found in all three kingdoms of life and catalyse carbon- or phosphoryl-transfer reactions [25] . The promiscuous substrate profiles and low levels of sequence similarity between HADs have made determining the in vivo function of many superfamily members difficult [26] . Within the HAD superfamily, PfHAD1 has the greatest sequence similarity to the Cof-like hydrolase subfamily (Interpro IPR000150) (ref. 27 ). This family is named for an Escherichia coli enzyme involved in thiamin biosynthesis [26] , [28] . Most members of the Cof subfamily are bacterial and most remain uncharacterized. Biochemical characterization suggests that members of this family utilize phosphorylated sugar substrates [26] , [29] . Sequence changes map to core and active site of PfHAD1 PfHAD1 changes found in FSM R strains map along the entire gene body ( Fig. 3a ). To define the structural basis for the role of these point mutations in PfHAD1 function, we solved the crystal structure of PfHAD1 to 2.05 Å ( Fig. 3b , Table 1 ). Clear electron density was not observed for the 6xHis tag in either chain, or the amino-terminal (N-terminal) region in chain B (residues 1–19), and were therefore not modelled. Like other members of the HAD superfamily, PfHAD1 consists of two distinct domains: a catalytic core domain (residues 1–106 and 212–288) and a cap domain (residues 107–211). The cap domain is inserted into the linker immediately following the third beta-strand. Table 1 Data collection and refinement statistics. Full size table The four sequence motifs required for the catalysis [25] of HAD superfamily members are structurally conserved in PfHAD1: motif I—DXD sequence at the end of strand I; motif II—a conserved threonine/serine at the end of strand II; motif III—a conserved lysine at the N terminus of the helix before strand IV; motif IV—a DD, GDxxxD or GDxxxxD on strand IV ( Fig. 3c ) [25] . The sequence 27-DLD-29 in PfHAD1 corresponds to motif I, Thr-61 corresponds to motif II, Lys-215 corresponds to motif III and the sequence 237-GDGEND-242 corresponds to the GDxxxD signature of motif IV. These structural motifs make up the substrate-binding site, located on the interface between the core and cap domains. These motifs are conserved among PfHAD1 homologues found in MEP pathway-containing organisms, including E. coli , Mycobacterium tuberculosis , the alga Chlamydomonas reinhardtii and Arabidopsis thaliana ( Fig. 3c ). Catalysis by PfHAD1 is metal–ion dependent, and the side chains of Asp-27 and Asp-238, and the backbone carbonyl oxygen of Asp-29, coordinate a magnesium ion in the structure ( Fig. 3c ). On the basis of homology to other HAD family phosphatases [25] , it is predicted that the phosphoryl group of sugar phosphate compounds binds by coordinating the magnesium ion and the side chains of Thr-61, Lys-215 and Asp-29. Asp-27 is predicted to perform nucleophilic attack of the phosphate group. As PfHAD1 was crystallized in the absence of a sugar phosphate substrate, a chloride ion occupies the likely phosphate-binding site based on structural similarity to other HAD sugar phosphatases. The point mutations identified in FSM R strains (T26R, G30E, A60E, W130R and Y148C) were mapped onto the PfHAD1 crystal structure ( Fig. 3b ). Trp-130 and Tyr-148 are located in a tightly packed hydrophobic inner region of the cap domain. Mutations of these aromatic residues to a charged arginine and a small polar cysteine residue, respectively, likely result in the misfolding of the cap domain. Similarly, Thr-26 and Ala-60 are located in the hydrophobic inner region of the core domain, and mutation of these residues to a charged glutamate and arginine, respectively, are predicted to result in the misfolding of the core domain. Finally, Gly-30 is located in the active site of PfHAD1, and a mutation to a glutamate with a much larger side chain is predicted to interfere with substrate binding. Together, the structural mapping of FSM R PfHAD1 mutations suggests that, similar to nonsense mutations, the FSM R nonsynonymous mutations result in the loss of function of PfHAD1 activity through drastic changes in the core or catalytic regions of PfHAD1. The N70S variant is not suspected to have changes in activity, as Asn-70 is located on the surface of PfHAD1 and away from the substrate-binding site. FSM R PfHAD1 alleles result in loss of phosphatase activity We next investigated the enzymatic activity of PfHAD1. Because PfHAD1 has sequence homology to known phosphatases [26] ( Fig. 3c ), we predicted that PfHAD1 is also a phosphatase. We expressed and purified recombinant wild-type PfHAD1, the N70S variant and three full-length variants (G30E, A60E and Y148C) found in FSM R strains. Recombinant PfHAD1 is active against a non-specific phosphatase substrate, para -nitrophenyl phosphate ( p NPP) ( Fig. 4 ). This compound has been used in phosphatase screens as an effective indicator of phosphatase activity [26] , [30] . Activity against p NPP is significantly reduced in each of the FSM R PfHAD1 variants ( Fig. 4 ). The N70S variant found in sequenced isolates has activity similar to the wild-type enzyme ( P =0.59, unpaired Student’s t -test). 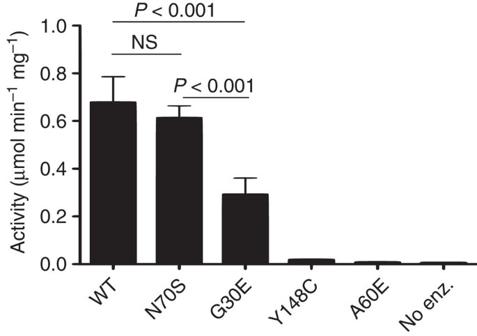Figure 4: PfHAD1 FSM-resistance alleles result in loss of phosphatase activity. Displayed are the means±s.e.m. of enzyme activity from at least three independent experiments.P-values were determined using a one-way analysis of variance (Tukey’s post test,α=0.05) in GraphPad Prism software. ‘NS’=not significant (P>0.05). ‘No enz.’=no enzyme. We were unable to obtain soluble T26R and W130R PfHAD1 variants. Figure 4: PfHAD1 FSM-resistance alleles result in loss of phosphatase activity. Displayed are the means±s.e.m. of enzyme activity from at least three independent experiments. P -values were determined using a one-way analysis of variance (Tukey’s post test, α =0.05) in GraphPad Prism software. ‘NS’=not significant ( P >0.05). ‘No enz.’=no enzyme. We were unable to obtain soluble T26R and W130R PfHAD1 variants. Full size image PfHAD1 complementation restores FSM sensitivity Because our FSM R strains are enriched for changes that result in loss of PfHAD1 function, we confirmed that restoring PfHAD1 expression would restore sensitivity to FSM. Using a piggyBac transposon system [31] , functional PfHAD1 was expressed in FSM R strain AM1, which possesses a premature truncation at amino acid 208 of the PfHAD1 locus and lacks detectable PfHAD1 ( Fig. 5a ). The expression construct produces green fluorescent protein (GFP)-tagged PfHAD1. The rescued strain, AM1 Hsp110:PfHAD1-GFP, retains its original mutation at the endogenous locus and successfully expresses PfHAD1-GFP. The expression pattern of Hsp110 is similar to that of PfHAD1 (ref. 32 ). The expression of functional PfHAD1 restores FSM sensitivity in AM1. While the FSM IC 50 of AM1 is 5.5±1.5 μM, AM1 Hsp110:PfHAD1-GFP has an IC 50 of 1.4±0.2 μM, similar to the parental IC 50 of 1.1±0.2 μM, indicating that loss of PfHAD1 function leads to FSM resistance in our strains ( Fig. 5b ). 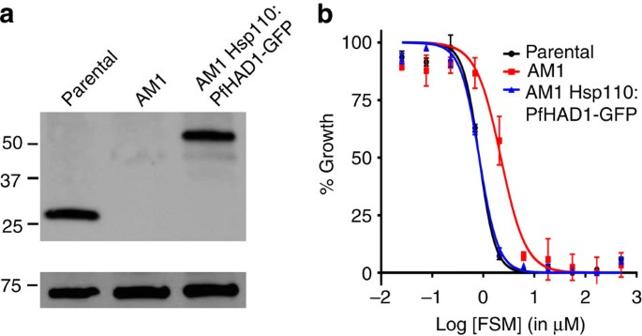Figure 5: Loss of PfHAD1 is required for FSM resistance. Data shown are representative of at least three independent experiments. (a) Immunoblot of the parent strain, FSMRstrain AM1 and AM1 Hsp110:PfHAD1-GFP. Full blots are shown inSupplementary Fig. 3. Marker units are kilodaltons (kDa). Top panel was probed with anti-PfHAD1 antisera, and the bottom panel was probed with anti-heat shock protein 70 (hsp70) antisera as a loading control. Expected approximate protein masses: native PfHAD1, 33 kDa; PfHAD1-GFP, 60 kDa; hsp70, 74 kDa. (b) FSM IC50s of the parent strain, FSMRstrain AM1, and AM1 Hsp110:PfHAD1-GFP. Displayed are the means±s.e.m. The parent strain has a FSM IC50of 1.1±0.2 μM, while AM1 has an IC50of 5.5±1.5 μM. Expression of PfHAD1-GFP in AM1 results in an IC50of 1.4±0.2 μM. Data shown are mean and are normalized such that 100% growth is defined by that of untreated cells and 0% growth is defined as the smallest value in each data set. Figure 5: Loss of PfHAD1 is required for FSM resistance. Data shown are representative of at least three independent experiments. ( a ) Immunoblot of the parent strain, FSM R strain AM1 and AM1 Hsp110:PfHAD1-GFP. Full blots are shown in Supplementary Fig. 3 . Marker units are kilodaltons (kDa). Top panel was probed with anti-PfHAD1 antisera, and the bottom panel was probed with anti-heat shock protein 70 (hsp70) antisera as a loading control. Expected approximate protein masses: native PfHAD1, 33 kDa; PfHAD1-GFP, 60 kDa; hsp70, 74 kDa. ( b ) FSM IC 50 s of the parent strain, FSM R strain AM1, and AM1 Hsp110:PfHAD1-GFP. Displayed are the means±s.e.m. The parent strain has a FSM IC 50 of 1.1±0.2 μM, while AM1 has an IC 50 of 5.5±1.5 μM. Expression of PfHAD1-GFP in AM1 results in an IC 50 of 1.4±0.2 μM. Data shown are mean and are normalized such that 100% growth is defined by that of untreated cells and 0% growth is defined as the smallest value in each data set. Full size image PfHAD1 is a sugar phosphatase Within the HAD superfamily, PfHAD1 has the greatest sequence similarity to the Cof-like hydrolase subfamily of sugar phosphatases. We assayed recombinant wild-type PfHAD1 with a number of phosphorylated sugar substrates ( Fig. 6 ). PfHAD1 has a wide substrate utilization profile and low substrate specificity, consistent with other members of this enzyme family [26] , [33] , [34] . PfHAD1 does not directly utilize FSM as a substrate. 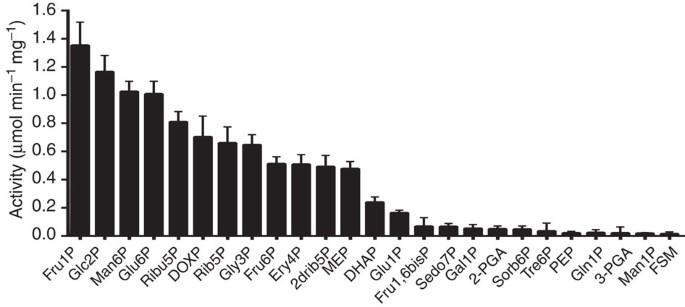Figure 6: PfHAD1 dephosphorylates sugar phosphates, including MEP pathway intermediates. Displayed are the means±s.e.m. of the enzyme activity from at least three independent experiments. DHAP, dihydroxyacetone phosphate; Ery4P, erythrose 4-phosphate; Fru1P, fructose 1-phosphate; Fru6P, fructose 6-phosphate; Fru1,6bisP, fructose 1,6-bisphosphate; Gal1P, galactose 1-phosphate; Glc2P, glycerol 2-phosphate; Gln1P, glucosamine 1-phosphate; Glu1P, glucose 1-phosphate; Glu6P, glucose 6-phosphate; Man1P, mannose 1-phosphate; Man6P, mannose 6-phosphate; PEP, phosphoenolpyruvate; Rib5P, ribose 5-phosphate; Ribu5P, ribulose 5-phosphate; Sedo7P, sedoheptulose 7-phosphate; Sorb6P, sorbitol 6-phosphate; Tre6P, trehalose 6-phosphate; 2drib5P, deoxyribose 5-phosphate; 2-PGA, 2-phosphoglyceric acid; 3-PGA, 3-phosphoglyceric acid. Figure 6: PfHAD1 dephosphorylates sugar phosphates, including MEP pathway intermediates. Displayed are the means±s.e.m. of the enzyme activity from at least three independent experiments. DHAP, dihydroxyacetone phosphate; Ery4P, erythrose 4-phosphate; Fru1P, fructose 1-phosphate; Fru6P, fructose 6-phosphate; Fru1,6bisP, fructose 1,6-bisphosphate; Gal1P, galactose 1-phosphate; Glc2P, glycerol 2-phosphate; Gln1P, glucosamine 1-phosphate; Glu1P, glucose 1-phosphate; Glu6P, glucose 6-phosphate; Man1P, mannose 1-phosphate; Man6P, mannose 6-phosphate; PEP, phosphoenolpyruvate; Rib5P, ribose 5-phosphate; Ribu5P, ribulose 5-phosphate; Sedo7P, sedoheptulose 7-phosphate; Sorb6P, sorbitol 6-phosphate; Tre6P, trehalose 6-phosphate; 2drib5P, deoxyribose 5-phosphate; 2-PGA, 2-phosphoglyceric acid; 3-PGA, 3-phosphoglyceric acid. Full size image In vitro , PfHAD1 is most active against monophosphorylated three to six-carbon monosaccharides, including intermediates of glycolysis, the pentose phosphate pathway and the MEP pathway ( Fig. 6 ). Kinetic parameters for the top three substrates as well as gly3P, a MEP pathway precursor, can be found in Supplementary Table 2 . The substrate profile of PfHAD1 is similar to that of related HADs in E. coli and A. thaliana [26] , [33] . Like other HADs, PfHAD1 dephosphorylates a variety of substrates in vitro . Catalytic efficiencies ( k cat / K m ) for the four measured substrates were within an order of magnitude and do not clearly indicate a preferred in vivo substrate, which is typical of this enzyme class. None of the purified recombinant FSM R PfHAD1 variants have significant activity against sugar phosphate substrates (maximum mean activity <0.9 μmol min −1 mg −1 for all variants against man6P, G6P, F6P, rib5P, gly3P and DHAP). PfHAD1 is localized to the cytoplasm MEP pathway enzymes are localized to the apicoplast in P. falciparum [14] , [35] . To help elucidate the mechanism by which PfHAD1 affects MEP pathway function, we examined the subcellular localization of PfHAD1. We raised specific polyclonal rabbit antisera against recombinant PfHAD1 and performed confocal immunofluorescence to localize PfHAD1. PfHAD1 is highly expressed in blood-stage parasites [36] . PfHAD1 appears to be cytoplasmic and has minimal overlap with the apicoplast marker ACP L -GFP (described by Waller, et al . [37] ; Fig. 7 ). Live fluorescent localization of PfHAD1-GFP (in strain AM1 Hsp110:PfHAD1-GFP) was similar to that of PfHAD1 immunolocalization in the fixed parental strain ( Supplementary Fig. 4 ). In addition, PfHAD1 lacks an apicoplast localization signal as predicted by the PlasmoAP and PATS algorithms [38] , [39] . Given the localization of PfHAD1, the enzyme likely utilizes phosphorylated sugars available in the cytoplasm, such as glycolytic intermediates. 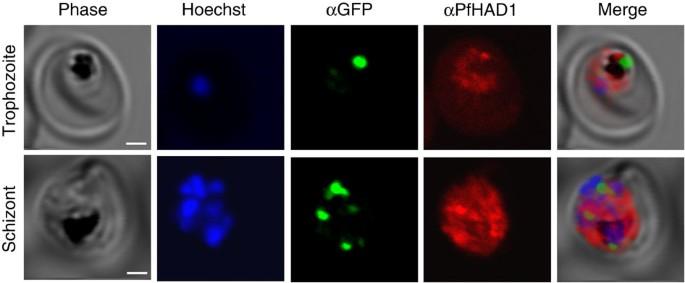Figure 7: PfHAD1 is expressed in blood-stage parasites and is localized to the parasite cytoplasm. Immunofluorescence confocal microscopy of ACPL-GFP trophozoite and schizont37, stained with αGFP and αPfHAD1 antibodies and Hoechst 33258 nuclear stain. Scale bars, 2 μm. Figure 7: PfHAD1 is expressed in blood-stage parasites and is localized to the parasite cytoplasm. Immunofluorescence confocal microscopy of ACP L -GFP trophozoite and schizont [37] , stained with αGFP and αPfHAD1 antibodies and Hoechst 33258 nuclear stain. Scale bars, 2 μm. Full size image FSM R strains increase levels of MEP pathway intermediates Since PfHAD1 dephosphorylates glycolytic intermediates, we predicted that the loss of PfHAD1 function would increase substrate availability to the MEP pathway, which requires gly3P and pyruvate. We evaluated the levels of MEP pathway intermediates in eight FSM R P. falciparum strains with PfHAD1 changes, using our previously described quantitative liquid chromatography-mass spectrometry method [8] ( Fig. 8 , Supplementary Table 3 ). Parental 3D7 and eight FSM R strains were treated +/− FSM for 10 h and the levels of MEP intermediates were quantified in each strain. Our method quantifies cellular levels of 1-deoxy-D-xylulose 5-phosphate (DOXP), 2-C-methylerythritol 4-phosphate (MEP), 4-diphosphocytidyl-2-C-methylerythritol and 2-C-methyl-D-erythritol 2,4-cyclopyrophosphate (MEcPP). 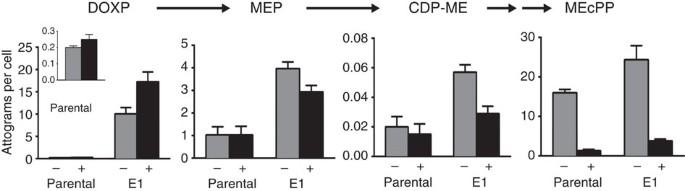Figure 8: Increased levels of MEP pathway intermediates in FSMRstrains with the loss of PfHAD1 function. Ring-stage parental and FSMRP. falciparumparasites were treated +/− 5 μM FSM for 10 h. Displayed are the means±s.e.m. of the metabolite levels from at least three independent experiments. Representative FSMRstrain E1 is shown, which possesses the K10XPfHAD1allele. The complete dataset is found inSupplementary Table 3. CDP-ME, 4-diphosphocytidyl-2-C-methylerythritol. Figure 8: Increased levels of MEP pathway intermediates in FSM R strains with the loss of PfHAD1 function. Ring-stage parental and FSM R P. falciparum parasites were treated +/− 5 μM FSM for 10 h. Displayed are the means±s.e.m. of the metabolite levels from at least three independent experiments. Representative FSM R strain E1 is shown, which possesses the K10X PfHAD1 allele. The complete dataset is found in Supplementary Table 3 . CDP-ME, 4-diphosphocytidyl-2-C-methylerythritol. Full size image FSM R strains with PfHAD1 mutations show an overall increase in levels of MEP pathway intermediates. Compared with the parental strain, FSM R strains have a 55.2±5.9-fold increase in the levels of DOXP, the substrate for PfDXR (median P <0.01, unpaired Student’s t -test). This increase is maintained during treatment with FSM (78.7±10.1-fold increase, median P <0.01; Fig. 8 , Supplementary Table 3 ) and would allow for DOXP to compete with FSM binding to PfDXR. Increased DOXP levels are not due to the increased transcript levels of PfDXS, the enzyme that produces DOXP ( Supplementary Fig. 2 ). FSM-treated FSM R strains also have an increase in MEcPP levels compared with the parental strain (2.7±0.43-fold, median P <0.01). In other systems, FSM resistance is due to the lack of FSM uptake or FSM efflux [40] , [41] , [42] . Metabolic profiling of FSM R parasites suggests that is not the mechanism of resistance in our strains. FSM treatment of FSM R strains results in metabolic changes that are still consistent with inhibition of PfDXR, the target of FSM. Specifically, the levels of the upstream metabolite DOXP increase, and levels of distal metabolites, such as MEcPP, decrease ( Fig. 8 , Supplementary Table 3 ) [8] . Our data are most consistent with a change in a metabolic regulator outside the MEP pathway that influences production of pathway intermediates, namely DOXP. In this study, we describe the genetic, biochemical, structural and metabolic basis for the resistance to the MEP pathway inhibitor FSM in the malaria parasite, Plasmodium falciparum. Our study represents a powerful use of next-generation sequencing to facilitate a forward genetics approach in a non-model organism to identify a new regulator of an essential biochemical pathway, the MEP pathway of isoprenoid biosynthesis. We identify a member of the HAD superfamily, PfHAD1, whose loss-of-function confers FSM resistance in P. falciparum . To our knowledge, PfHAD1 is the first cellular factor that regulates the MEP pathway in P. falciparum . PfHAD1 has structural similarity to other members of the HAD superfamily, retains the motifs necessary for catalysis, and is active against sugar phosphates. Loss of PfHAD1 function causes dramatically increased levels of MEP pathway metabolites, particularly DOXP, the substrate of DXR. Our work suggests a model of PfHAD1 function, shown in Fig. 9 . We propose that PfHAD1 is a negative regulator of the MEP pathway. It typically catalyses the dephosphorylation of cytosolic phosphometabolites, such as glycolytic intermediates, to decrease the availability of substrates to the MEP pathway. Loss of sugar phosphatase activity in FSM R malaria parasites results in increased pools of DOXP, which overcomes competitive inhibition of PfDXR by FSM. 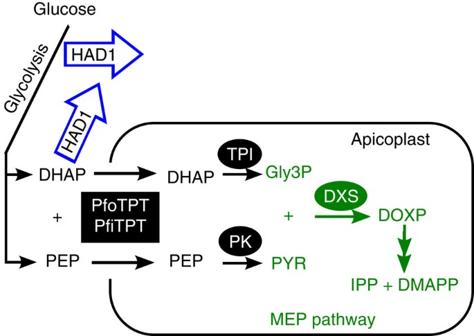Figure 9: Model of PfHAD1 function. PfHAD1 (blue arrows) may dephosphorylate the intermediates of glycolysis. Loss of PfHAD1 may increase local levels of sugar phosphates and increase the substrate availability to the apicoplast MEP pathway (green). The use of PEP as a substrate is unlikely, given the poor PfHAD1 activity against this substratein vitro(Fig. 6). Green reactions and substrates are part of the MEP pathway. PfiTPT and PfoTPT are transporters responsible for the import of PEP and DHAP into the apicoplast56,57. The conversion of PEP and DHAP into pyruvate and gly3P, respectively, are catalysed by apicoplast-localized pyruvate kinase (PK)58and triosephosphate isomerase (TPI)59. DHAP, dihydroxyacetone phosphate; DMAPP, dimethylallyl pyrophosphate; IPP, isopentenyl pyrophosphate; PEP, phosphoenolpyruvate. Figure 9: Model of PfHAD1 function. PfHAD1 (blue arrows) may dephosphorylate the intermediates of glycolysis. Loss of PfHAD1 may increase local levels of sugar phosphates and increase the substrate availability to the apicoplast MEP pathway (green). The use of PEP as a substrate is unlikely, given the poor PfHAD1 activity against this substrate in vitro ( Fig. 6 ). Green reactions and substrates are part of the MEP pathway. PfiTPT and PfoTPT are transporters responsible for the import of PEP and DHAP into the apicoplast [56] , [57] . The conversion of PEP and DHAP into pyruvate and gly3P, respectively, are catalysed by apicoplast-localized pyruvate kinase (PK) [58] and triosephosphate isomerase (TPI) [59] . DHAP, dihydroxyacetone phosphate; DMAPP, dimethylallyl pyrophosphate; IPP, isopentenyl pyrophosphate; PEP, phosphoenolpyruvate. Full size image FSM R malaria strains are highly enriched for genetic changes in the PfHAD1 locus. In our study, we identified 11 separate deleterious genotypic changes in PfHAD1 . If FSM is approved for clinical use, these changes may represent the genetic biomarkers of FSM resistance. While other genetic changes are also present in the FSM R strains ( Supplementary Data 1 ), our data indicate that the loss of PfHAD1 is the primary driver of resistance. In addition, changes in PfHAD1 genotype correlate not only with FSM resistance, but also with increased cellular levels of isoprenoid precursor metabolites. Complementation of a deleterious PfHAD1 allele restores FSM sensitivity. These findings strongly support that the primary biochemical change responsible for these phenotypes is the loss of PfHAD1 function. PfHAD1 is a member of the large, diverse HAD superfamily of aspartate nucleophile hydrolases, and belongs to the subfamily of Cof-like hydrolases (Interpro IPR00150). Many HAD family members have been structurally and enzymatically characterized [26] , [29] , [33] , [34] . However, the cellular functions of this group of enzymes are largely unknown. The Cof-like hydrolases are absent from animal and fungal genomes, but are highly expanded in bacteria. In addition, Cof-like hydrolases are uniformly present in eukaryotes that possess a plastid-like organelle, such as chloroplast-containing plants, and the apicomplexan parasites, such as P. falciparum . This phylogeny parallels that of the MEP pathway, which is also exclusive to many bacteria and plastid-containing eukaryotes, and absent in animals or fungi. Since few studies have addressed the potential biological function of these enzymes, additional work is required to determine whether PfHAD1 homologues represent regulators of isoprenoid biosynthesis in other MEP pathway-containing organisms. Evidence suggests that this may be the case in bacteria, since the E. coli PfHAD1 ortholog YidA was identified in a colorimetric screen of E. coli for increased lycopene production [43] . During its intraerythrocytic development cycle, glycolysis is the primary source for ATP generation in P. falciparum [44] . As a result, the malaria parasite has great capacity for glucose uptake and carbon flux through glycolysis. PfHAD1 has a broad substrate profile, and readily dephosphorylates a range of three to six-carbon monophosphorylated substrates, including glycolytic and pentose phosphate intermediates, as well as MEP pathway metabolites. Given this promiscuity, it is unclear which metabolite/s represent the natural in vivo substrate/s for PfHAD1 and other Cof-like subfamily members. Thus, our studies do not distinguish which upstream metabolic step is regulated by PfHAD1. In addition, it is unclear why malaria parasites produce an enzyme whose activity would decrease glycolysis and ATP production. Genetic conservation of PfHAD1 in clinical and laboratory isolates of P. falciparum , as well as among PfHAD1 homologues in divergent organisms, suggests that these proteins have important cellular functions under typical growth conditions. The MEP pathway is an important target for the development of small-molecule inhibitors, since this pathway is absent in animals but essential in plants and key human pathogens, including malaria parasites and M. tuberculosis . Our studies highlight what may be a particular challenge in developing novel MEP pathway inhibitors. Even though FSM R strains are capable of growth in the presence of FSM, drug treatment still substantially reduces levels of the distal MEP pathway metabolite, MEcPP. Following FSM treatment, MEcPP levels in FSM R strains are reduced to ~20% of the concentrations present in untreated, wild-type parasites. This suggests that, at least in malaria parasites, cells direct more flux through the MEP pathway than is absolutely required for development, and therefore, they are capable of growth even when MEP pathway metabolism is substantially reduced. As novel MEP pathway inhibitors are developed, it appears that these compounds must achieve a sobering near-complete inhibition of the cellular MEP pathway in order to inhibit malaria parasite growth. Reagents Reagents were purchased from Sigma-Aldrich unless otherwise indicated. Maintenance of P. falciparum cultures The P. falciparum strain used for FSM selection is derived from genome reference strain 3D7 (ref. 45 ). The ACP L -GFP (expresses apicoplast-targeted GFP) strain used for immunofluorescence microscopy is described in Waller, et al . [37] . 3D7 and ACP L -GFP were obtained from the Malaria Research and Reference Reagent Resource Center (strains MRA-102 and MRA-568, respectively, MR4, ATCC, Manassas, Virginia). Unless otherwise stated, P. falciparum strains were cultured at 37 °C in a 2% suspension of human erythrocytes in RPMI-1640 medium (Sigma-Aldrich, SKU R4130) supplemented with 27 mM sodium bicarbonate, 11 mM glucose, 5 mM HEPES, 1 mM sodium pyruvate, 0.37 mM hypoxanthine, 0.01 mM thymidine, 10 μg ml −1 gentamycin and 0.5% albumax (Life Technologies) in a 5% O 2 /5% CO 2 /90% N 2 atmosphere, as previously described [8] , [46] . Culture growth was monitored by microscopic analysis of Giemsa-stained blood smears. Generation of FSM R P. falciparum A 3D7 parental strain was cloned by limiting dilution and used as the parental strain for all selections. Independent selections are defined as those cultures that were cultured in separate wells before and during selection. The parental strain was at 4% parasitemia in 4-ml cultures at the initiation of FSM selection. Parasites were initially cultured in media containing 0.5–1 μM FSM and gradually scaled to final concentrations of 2–4 μM FSM. The following FSM R strains were cloned by limiting dilution: E1, D6, MK1, D3, AM1 and AM2. Quantification of FSM resistance Asynchronous P. falciparum cultures were diluted to 1% parasitemia and were treated with FSM (Life Technologies) at concentrations ranging from 0.025–500 μM. Growth inhibition assays were performed in opaque 96-well plates at 100 μl culture volume. After 3 days, parasite growth was quantified by measuring DNA content using Picogreen (Life Technologies), as previously described [47] . Picogreen fluorescence was measured on a FLUOstar Omega microplate reader (BMG Labtech) at 485 nm excitation and 528 nm emission. IC 50 values were calculated by nonlinear regression analysis using GraphPad Prism software. Whole genome sequencing and variant discovery Genomic DNA was isolated from P. falciparum cells by a standard phenol-chloroform extraction and ethanol precipitation protocol [48] . Sequencing libraries were prepared and sequenced by the Washington University Genome Technology Access Center (GTAC). Briefly, 5 μg of genomic DNA was sheared to an average size of 175 bp. Fragments were end repaired and an ‘A’ base was added to the 3′ end. Adapters containing index sequences were ligated to the fragments. Resulting libraries were sequenced on an Illumina HiSeq 2000 to obtain 101 bp paired end reads. Bioinformatic analyses were performed by GTAC. Reads were not merged, but were aligned to the P. falciparum reference genome using Novoalign (Novocraft Technologies). PCR duplicates were removed using Picard and variants were analysed using SAMtools. SNPs were called if present in >50% of the reads. For all samples, at least 75% of coding regions were sequenced at ⩾ 5 × coverage. All whole genome sequencing data is available in the NCBI BioProject database and Sequence Read Archive. Sanger sequencing of PfHAD1 The region of interest was amplified from P. falciparum genomic DNA using the following gene-specific primers: 5′-GGTTCAAGGGTGATAGATAGGA-3′, 5′-CGAAGGTCCAACATAAGCAG-3′, 5′-ATGCACGAAATTGTAGATAAGAATG-3′, 5′-AATTCATGTATCTCCATTTTCAAGTC-3′ and 5′-GATCACTACATTTTGGACGTACAC-3′. Purified PCR products were sequenced by the Washington University Protein and Nucleic Acid Laboratory using BigDye Terminator v3.1 Cycle Sequencing reagents (Life Technologies). Chromatogram files were analysed using DNAStar SeqMan software. Representative traces for all strains are available through the NCBI Trace Archive. Recombinant expression and purification of PfHAD1 variants All PfHAD1 (PlasmoDB ID PF3D7_1033400) alleles were amplified from P. falciparum genomic DNA using the following primers: 5′–CTCACCACCACCACCACCATATGCACGAAATTGTAGATAAGAA-3′ and 5′- ATCCTATCTTACTCACTTATATGTCACAGAATGTCTTCA-3′. The PCR product was cloned by ligation-independent cloning into vector BG1861 (ref. 49 ), which introduces an N-terminal 6xHis tag and the construct was verified by Sanger sequencing. BG1861:6xHis-PfHAD1 was transformed into BL21(DE3)pLysS Escherichia coli cells (Life Technologies). Following induction with isopropyl-β-D-thiogalactoside, cells were collected by centrifugation and stored at −20 °C. Pellets were resuspended in lysis buffer containing 10 mM Tris HCl (pH 7.5), 20 mM imidazole, 01 mM MgCl 2 , 01 mM dithiothreitol, 1 mg ml −1 lysozyme, 100 U benzonase and Complete Mini EDTA-free protease inhibitor tablets (Roche Applied Science). 6xHis-PfHAD1 was bound to nickel agarose beads (Gold Biotechnology), eluted in 300 mM imidazole, 20 mM Tris HCl (pH 7.5) and 150 mM NaCl, and dialyzed in buffer lacking imidazole before analysis. Protein was flash frozen and stored at −80 °C. Crystallization and structure determination PfHAD1 was further purified by gel chromatography using a HiLoad 16/600 Superdex 200 pg column (GE Healthcare) equilibrated with 10 mM Tris (pH 8.0), 150 mM NaCl and 5 mM dithiothreitol. The fractions containing PfHAD1 were pooled and concentrated to 20 mg ml −1 using a centrifugal filter. Crystals of PfHAD1 were obtained by vapour diffusion using hanging drops equilibrated at 18 °C against 500 μl of a reservoir containing 0.1 M HEPES (pH 7.5) and 20–25% PEG 8000. Crystals were cryo-protected with 0.1 M HEPES (pH 7.5) and 30% PEG 8000 before flash-freezing under liquid nitrogen for data collection. X-ray data were collected from a single crystal using a wavelength of 1 Å at synchrotron beamline 4.2.2 of the Advanced Light Source in Berkeley, CA. Data were processed with XDS [50] and the coordinates from PDB 2B30 were used as a search model for phase determination by molecular replacement using PHENIX [51] . Rigid-body refinement followed by automatic model rebuilding were performed in PHENIX [51] . Subsequent iterated manual building/rebuilding and refinement of models were performed using Coot [52] and PHENIX [51] , respectively. The structure validation server MolProbity [53] was used to monitor refinement. The final refined model results in a Ramachandran plot with 96.75% of residues in the favored region and 3.25% in the allowed region. A complete summary of the final crystallographic refinement statistics are given in Table 1 and a stereo image of a representative region of the electron density map is shown in Supplementary Fig. 5 . Figures were prepared using PyMOL Molecular Graphics System, Version 0.99rc6, Schrödinger, LLC. Structure data is deposited in the RSCB Protein Structure Database. pTEOE110:PfHAD1-GFP plasmid construction The construct used to express PfHAD1 in FSM R strains, pTEOE110, was a gift from Daniel Goldberg (Washington University, St. Louis). The construct contains the heat shock protein 110 (PF3D7_0708800) 5′ UTR [54] and a carboxyl-terminal GFP tag. The human dihydrofolate reductase selectable marker confers resistance to WR92210. These sites are flanked by inverted terminal repeats [31] that allow for integration of the segment containing the Hsp110 5′ UTR, the gene of interest, GFP and human dihydrofolate reductase into the genome, facilitated by a co-expression from a plasmid encoding the piggyBac transposase (pHTH, MRA912, MR4, ATCC, Manassas, Virginia). PfHAD1 was amplified using the following primers: 5′-CATGCTCGAGATGCACGAAATTGTAGATAAGAA-3′ and 5′-CATGCCTAGGTATGTCACAGAATGTCTTCAAG-3′. The resulting PCR product was cloned into the XhoI and AvrII sites in pTEOE110 to generate pTEOE:PfHAD1. Successful insertion was confirmed by colony PCR and Sanger sequencing. P. falciparum transfection Seventy-five micrograms of each plasmid (pTEOE110:PfHAD1 and pHTH) was combined, precipitated and resuspended in 400 μl Cytomix (120 mM KCl, 0.15 mM CaCl 2 , 2 mM EGTA, 5 mM MgCl 2 , 10 mM K 2 HPO 4 , 25 mM HEPES, pH 7.6). A 4-ml culture of FSM R strain AM1 was synchronized by treatment with 5% sorbitol to obtain ring-stage parasites at >4% parasitemia. Cells were washed with Cytomix and resuspended in 400 μl DNA/Cytomix solution. Cells were electroporated using a Biorad GenePulser II electroporator set to 950 μF capacitance and 0.31 kV. Transfected cells were washed with media and returned to the previously described culture conditions. Culture media was replaced daily for one week. Cultures were maintained under selection with 5 nM WR92210 (Jacobus Pharmaceutical Co.) beginning 48 h post transfection. Parasite growth was monitored by microscopy. Successful transfectants were cloned by limiting dilution. The resulting strain was verified by microscopy, western blot and sequencing of the endogenous PfHAD1 locus. Generation of PfHAD1 polyclonal antisera PfHAD1 rabbit polyclonal antisera was produced by Cocalico Biologicals (Reamston, PA) using their standard protocol. Purified recombinant 6XHis-PfHAD1 was used as an antigen. Titermax was used as an adjuvant. Immunoblotting P. falciparum cells were obtained by treatment of infected erythrocytes with 0.1% saponin. Lysates were separated on a polyacrylamide gel and transferred to polyvinylidene fluoride membrane. For the detection of PfHAD1, the membrane was blocked and probed with 1:20,000 anti-PfHAD1 polyclonal antisera (Cocalico Biologicals), followed by 1:20,000 HRP-conjugated goat anti-rabbit IgG polyclonal antibody (Life Technologies). The membrane was stripped by treatment with 200 mM glycine, 0.1% sodium dodecyl sulphate, 1% Tween-20 (pH 2.2) and reprobed with 1:5,000 anti-heat shock protein 70 antibody (Agrisera) as a loading control. Enzymatic assays All assays were performed in clear 96-well half-area plates using a FLUOstar Omega microplate reader (BMG Labtech) at 37 °C. Reaction rates were determined using GraphPad Prism software. Phosphatase activity was measured using the substrate p NPP (New England Biolabs). Reactions were performed in 50 μl volumes with 10 mM p NPP, 50 mM Tris HCl (pH 7.5), 5 mM MgCl 2 and 0.5 mM MnCl 2 . Reactions contained 2 μg purified recombinant enzyme. Para -nitrophenyl production was quantified by absorbance at 405 nm. Enzyme activity against phosphorylated sugar substrates was measured using the Enzchek Phosphate Assay Kit (Life Technologies) according to supplier instructions. Each assay contained 200 ng recombinant purified enzyme and 1 mM substrate. Substrates were purchased from Sigma-Aldrich, except for DOXP and MEP (Echelon Biosciences), fructose 1-phosphate (Santa Cruz Biotechnology) and FSM (Life Technologies). For the determination of kinetic parameters, assays were performed using 50 ng 6XHis-PfHAD1 and 0.03–12 mM substrate. Data were fit to Michaelis–Menten curves using GraphPad Prism software. Microscopy For immunofluorescence microscopy, cells at ~10% parasitemia were fixed in 4% paraformaldehyde in PBS. Fixed cells were washed with 50 mM ammonium chloride, permeabilized by treatment with 0.075% NP-40 in PBS and blocked using 2% bovine serum albumin. Cells were incubated with the following antibody dilutions: 1:10,000 rabbit polyclonal anti-PfHAD1 (described above) and 1:1,000 mouse monoclonal anti-GFP (Life Technologies #A11120) for the detection of GFP in the ACP L -GFP strain (MRA-568). Hoechst 33258 (Life Technologies) was used as a nuclear counterstain. Secondary antibodies used were 1:200 dilutions of Alexa Fluor 568 goat anti-rabbit IgG (Life Technologies #A11011) and Alexa Fluor 488 goat anti-mouse IgG (Life Technologies #A11029). Images were obtained on an Olympus Fluoview FV1000 confocal microscope. For imaging of live cells, cells were stained with 10 ng μl −1 Hoechst 33258 for 10 min and mounted under coverslips on polysine adhesion slides. Cells were visualized on an Olympus BH8 microscope at room temperature for no longer than 15 min. For all microscopy, minimal adjustments in brightness and contrast were applied equally to all images. Sample preparation for mass spectrometry analysis P. falciparum were cultured in 75 ml volumes in 150 × 25 mm tissue culture dishes at 4% haematocrit until >6% parasitemia was reached. Cultures were synchronized by one to two treatments with 5% sorbitol until >8% parasitemia and >75% of parasites were in ring-stage growth. Once these criteria were met, 75 ml cultures were split into 3 × 25 ml samples. Ring-stage cultures were then treated +/− 5 μM FSM (Life Technologies) for either 0 or 10 h. At each time point, parasite-infected erythrocytes were lysed with 0.1% saponin, the parasite pellets washed with PBS and the pellets stored at −80 °C until extraction. Samples were extracted and analysed by liquid chromatography-mass spectrometry as previously described [8] . Briefly, samples were extracted in chloroform, methanol and acetonitrile (2:1:1, v/v/v) and homogenized. Water was added and the sample was homogenized again. The polar phase was separated by centrifugation, lyophilized and resuspended in water for analysis. Quantitative PCR of PfDXS and PfDXR transcripts Infected erythrocytes were lysed by treatment with 0.1% saponin. Parasite pellets were stored at −80 °C until extraction. Total RNA was isolated using the Ambion Purelink RNA Mini kit (Life Technologies) according to the supplier’s instructions. After the first wash step, samples underwent an on-column DNase treatment (Qiagen) for 30 min. RNA was eluted in RNase-free water, quantified and stored at −80 °C until further use. At least 100 ng of RNA was used to synthesize cDNA using the Quantitect Reverse Transcription kit (Qiagen), according to the supplier’s instructions. Amplification of cDNA was performed using an Applied Biosystems Fast RT PCR System and Applied Biosystems Fast SYBR Green PCR Master Mix (Life Technologies). PfDXS (PlasmoDB ID PF3D7_1337200) was amplified using the following primers: 5′-AACGTGGATAAAGTACACATTGC-3′ and 5′-TGATATACTTACGGCATTTGTTGG-3′ and PfDXR (PlasmoDB ID PF3D7_1467300) was amplified using the following primers; 5′- ACATGGCCTGATAGAATAAAAACA-3′ and 5′- TTCATTTGACGCATTTAGTACAGTT-3′ (Sigma-Aldrich). The gene encoding beta tubulin (PF3D7_1008700) was used as a control and was amplified using the following primers: 5′-ATCCCATTCCCACGTTTACATT-3′ and 5′-TCCTTTGTGGACATTCTTCCTC-3′ (Eurofins MWG Operon). Standard curves were used to verify primer efficiency (r 2 >0.97, E >80%). In addition to SYBR Master Mix, reactions contained 10 ng cDNA and 300 nM of each primer. All reactions were performed in MicroAmp Fast Optical 96-well plates (Life Technologies). Thermocycling parameters were as follows: 95 °C for 30 s, 40 cycles of 95 °C for 3 s and 60 °C for 30 s. Agarose gel electrophoresis, as well as melt-curve analysis, with temperatures ranging from 60 to 95 °C, confirms production of a single product from each primer pair. Controls lacking either reverse transcriptase or template produced no significant signals. C t values were generated using 7500 Fast System software (Applied Biosystems). Relative PfDXS and PfDXR expression levels were calculated using the ΔΔ C t method. Δ C t values were calculated by subtracting the C t of the reference gene (beta tubulin) from the target gene ( PfDXS or PfDXR ). ΔΔ C t values were then calculated by normalizing to the Δ C t of the parental sample. Relative expression changes were calculated as 2 −ΔΔ C t . How to cite this article: Guggisberg, A. M. et al . A sugar phosphatase regulates the methylerythritol phosphate (MEP) pathway in malaria parasites. Nat. Commun. 5:4467 doi: 10.1038/ncomms5467 (2014). Accession codes: Whole genome sequences of parental, FSM R , and control strains have been deposited in the NCBI BioProject Database and Sequence Read Archive under accession codes PRJNA222697 and SRP038937 , respectively. Representative Sanger sequencing traces verifying PfHAD1 SNPs have been deposited in the NCBI Trace Archive under accession codes 2338198460 to 2338198575. PfHAD1 protein structure data has been deposited in the RCSB Protein Data Bank under accession code 4QJB .